TRPM2 links oxidative stress to NLRP3 inflammasome activation Exposure to particulate crystals can induce oxidative stress in phagocytes, which triggers NLRP3 inflammasome-mediated interleukin-1β secretion to initiate undesirable inflammatory responses that are associated with both autoinflammatory and metabolic diseases. Although mitochondrial reactive oxygen species have a central role in NLRP3 inflammasome activation, how reactive oxygen species signal assembly of the NLRP3 inflammasome remains elusive. Here, we identify liposomes as novel activators of the NLRP3 inflammasome and further demonstrate that liposome-induced inflammasome activation also requires mitochondrial reactive oxygen species. Moreover, we find that stimulation with liposomes/crystals induced reactive oxygen species-dependent calcium influx via the TRPM2 channel and that macrophages deficient in TRPM2 display drastically impaired NLRP3 inflammasome activation and interleukin-1β secretion. Consistently, Trpm2 −/− mice are resistant to crystal-/liposome-induced interleukin-1β-mediated peritonitis in vivo . Together, these results identify TRPM2 as a key factor that links oxidative stress to the NLRP3 inflammasome activation. Therefore, targeting TRPM2 may be effective for the treatment of NLRP3 inflammasome-associated inflammatory disorders. Liposomes are particles consisting of self-aggregated lipids and are commonly used as effective immune adjuvants and efficient drug-delivery vehicles to treat various infectious and cancerous diseases [1] , [2] , [3] , [4] . Although previous studies have indicated that liposomes can enhance the expression of chemokines, such as CCL2, and co-stimulatory molecules, such as CD80/86, in antigen-presenting cells [5] , [6] , [7] , [8] , little is known about whether an innate immune receptor exists to sense the presence of liposomes. During the past decade, a number of studies have demonstrated that particulate substances such as alum, silica, monosodium urate and calcium pyrophosphate dihydrate crystals can induce NLRP3 (nod-like receptor family, pyrin domain containing 3) inflammasome activation, which mediates the secretion of biologically active interleukin-1β (IL-1β) from macrophages [9] , [10] , [11] , [12] , [13] . As liposomes are also particulate in nature, we hypothesized that the NLRP3 inflammasome may serve as an innate immune sensor for liposomes. Although the precise mechanism by which the NLRP3 inflammasome is activated remains unknown, several stress-related cellular processes, including cytosolic depletion of potassium, lysosome disruption, mitochondrial damage and intracellular calcium elevation, have been proposed to be involved in the activation of this inflammasome [14] , [15] . Mitochondria are an ancient and evolutionarily conserved cellular organelle that have a key role in regulating the signalling pathways of pattern recognition receptors [16] , including the NLRP3 inflammasome. Upon stimulation with particulate stimuli, mitochondria can transmit stress signals to alarm the immune system via secondary signalling messengers, such as mitochondrial reactive oxygen species (ROS) [16] , [17] , [18] . Blocking ROS generation by mitochondria has been shown to abolish NLRP3 inflammasome activation whereas artificial induction of mitochondrial ROS can spontaneously induce NLRP3-mediated IL-1β secretion [19] , [20] . Although it is clear that mitochondrial ROS have a pivotal role, the precise mechanism underlying ROS-induced NLRP3 inflammasome activation remains poorly understood. In this study, we identified liposomes as a novel group of particulate activators of the NLRP3 inflammasome and further demonstrated that liposomes/crystals induced mitochondrial ROS production, which subsequently triggered a calcium influx via the plasma membrane cation channel TRPM2 (transient receptor potential melastatin 2). Notably, TRPM2 deficiency dramatically impaired liposome-/crystal-induced NLRP3 inflammasome activation, bioactive IL-1β release and subsequent inflammatory responses. These observations identify a novel role for TRPM2 in linking oxidative stress to calcium mobilization, which ultimately results in NLRP3 inflammasome activation. Liposomes induce NLRP3 inflammasome-dependent IL-1β release It is generally accepted that a ‘two-step’ process is necessary for NLRP3 inflammasome-mediated IL-1β release. The first step requires NF-κB activation to induce synthesis of pro-IL-1β, whereas the second step involves assembly of a large cytosolic protein complex, termed inflammasomes, which lead to caspase-1 activation. Caspase-1 then cleaves pro-IL-1β into its mature form [21] . To determine whether liposomes can trigger activation of the NLRP3 inflammasome, we first tested whether several liposomes, consisting of different phospholipids, can induce bioactive IL-1β release in macrophages. Cationic (DOTAP, DC-Chol and DDA) and anionic (DPPC-DMPG) liposomes elicited IL-1β release from lipopolysaccharide (LPS)-primed murine bone marrow-derived macrophages (BMDMs) and phorbol 12-myristate 13-acetate (PMA)-primed human THP-1 cells ( Fig. 1a ), and the levels of secreted IL-1β were dependent on the dose and size of the liposomes ( Supplementary Fig. S1 ). Procaspase-1 was autocleaved after stimulation with charged liposomes, and active caspase-1 was responsible for the maturation of IL-1β ( Fig. 1c ). Unlike IL-1β release, the secretion of both tumour-necrosis factor (TNF) and IL-6, which relies on NF-κB activation, was not enhanced in LPS-primed BMDMs after liposomes stimulation ( Supplementary Fig. S2a,b ). Consistently, liposomes alone did not induce either TNF or IL-6 secretion in unprimed macrophages ( Supplementary Fig. S2c ). In sharp contrast to the charged liposomes, neutral liposomes, such as DOPC and PC-Chol liposomes, failed to trigger IL-1β secretion ( Fig. 1a and Supplementary Fig. S3a,b ). However, the incorporation of cationic lipids into neutral liposomes rescued IL-1β secretion ( Supplementary Fig. S3c ), which suggests that the charge of liposomes determines their ability to induce IL-1β release. Furthermore, although liposomes induced low levels of cytotoxicity in macrophages ( Supplementary Fig. S4 ), ATP and uric acid, two known NLRP3 inflammasome agonists that are released from dying cells [13] , [22] , were not intermediates responsible for liposome-induced IL-1β secretion ( Supplementary Fig. S5 ). 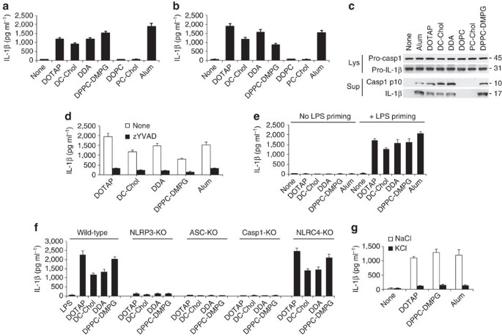Figure 1: Charged liposomes activate the NLRP3 inflammasome to induce IL-1β secretion. ELISA for IL-1β from the supernatants of (a) LPS-primed wild-type BMDMs or (b) PMA-primed THP1 cells that were stimulated with either the indicated liposomes (30 μg ml−1for BMDMs and 50 μg ml−1for THP1 cells) or alum (250 μg ml−1for BMDMs and 500 μg ml−1for THP1 cells). (c) Immunoblots of procaspase-1, activated caspase-1 (p10), pro-IL-1β and cleaved IL-1β (p17) in the culture supernatants (Sup) and cell lysates (Lys) from LPS-primed BMDMs after stimulation with indicated liposomes or alum. (d) IL-1β from supernatants of LPS-primed BMDMs that were pretreated with caspase-1 inhibitor (z-YVAD-fmk, 10 μM) for 45 min followed by stimulations with indicated liposomes or alum. (e) ELISA for IL-1β from the supernatants of LPS-primed or unprimed wild-type BMDMs that were stimulated with indicated liposomes (30 μg ml−1) or alum (250 μg ml−1). (f) The IL-1β levels from the supernatants of LPS-primed immortalized mouse macrophages from wild-type,Nlrp3−/−,Asc−/−, Caspase-1−/−orNlrc4−/−mice that were stimulated with liposomes (70 μg ml−1). (g) ELISA for IL-1β from the supernatants of LPS-primed wild-type BMDMs that were cultured in 150 mM of KCl or NaCl followed by stimulation with liposomes or alum. Data in (a,b,d–g) are shown as mean±s.d., and all data are representative of at least three independent experiments. Figure 1: Charged liposomes activate the NLRP3 inflammasome to induce IL-1β secretion. ELISA for IL-1β from the supernatants of ( a ) LPS-primed wild-type BMDMs or ( b ) PMA-primed THP1 cells that were stimulated with either the indicated liposomes (30 μg ml −1 for BMDMs and 50 μg ml −1 for THP1 cells) or alum (250 μg ml −1 for BMDMs and 500 μg ml −1 for THP1 cells). ( c ) Immunoblots of procaspase-1, activated caspase-1 (p10), pro-IL-1β and cleaved IL-1β (p17) in the culture supernatants (Sup) and cell lysates (Lys) from LPS-primed BMDMs after stimulation with indicated liposomes or alum. ( d ) IL-1β from supernatants of LPS-primed BMDMs that were pretreated with caspase-1 inhibitor (z-YVAD-fmk, 10 μM) for 45 min followed by stimulations with indicated liposomes or alum. ( e ) ELISA for IL-1β from the supernatants of LPS-primed or unprimed wild-type BMDMs that were stimulated with indicated liposomes (30 μg ml −1 ) or alum (250 μg ml −1 ). ( f ) The IL-1β levels from the supernatants of LPS-primed immortalized mouse macrophages from wild-type, Nlrp3 −/− , Asc −/− , Caspase-1 −/− or Nlrc4 −/− mice that were stimulated with liposomes (70 μg ml −1 ). ( g ) ELISA for IL-1β from the supernatants of LPS-primed wild-type BMDMs that were cultured in 150 mM of KCl or NaCl followed by stimulation with liposomes or alum. Data in ( a , b , d – g ) are shown as mean±s.d., and all data are representative of at least three independent experiments. Full size image Next, we sought to determine whether the intact NLRP3 inflammasome machinery was essential for liposome-induced IL-1β secretion. First, we observed that liposome-induced IL-1β secretion required LPS priming ( Fig. 1e ). Moreover, macrophages deficient in NLRP3, ASC or caspase-1, three key components of the NLRP3 inflammasome, all failed to respond to liposome stimulation after LPS priming ( Fig. 1f ). In contrast, macrophages deficient in NLRC4, another Nod-like receptor that recognizes bacterial flagellin [23] , or AIM2 (absence in melanoma 2), an immune sensor for DNA [24] , [25] , responded to charged liposomes stimulation in a manner similar to wild-type cells ( Fig. 1f and Supplementary Fig. S6 ). These data collectively suggest that charged liposomes induced IL-1β secretion specifically via activation of the NLRP3 inflammasome. To further confirm that charged liposomes activate the NLRP3 inflammasome, we next tested whether potassium efflux, a seemingly obligatory event during NLRP3 inflammasome activation [14] , [21] , [26] , was necessary for liposome-induced inflammasome activation. Indeed, the blockade of potassium efflux with a high concentration of KCl drastically decreased the liposome-induced NLRP3 inflammasome activation ( Fig. 1g ). Similar results were also obtained when glibenclamide, an inhibitor that blocks potassium channels [27] , was used (data not shown). Hereafter, we used DOTAP and DPPC-DMPG liposomes as the representative cationic and anionic liposomes, respectively, to investigate the mechanism by which charged liposomes activate the NLRP3 inflammasome. NLRP3 inflammasome activation requires uptake of liposomes NLRP3 is a cytosolic innate immune receptor that, upon activation, recruits ASC and procaspase-1 to assemble into the inflammasome [26] . Therefore, we next tested whether cellular uptake of liposomes was necessary for activation of the NLRP3 inflammasome. The inhibition of the endocytic pathway with cytochalasin D, a potent inhibitor of actin polymerization [12] , greatly reduced liposome-induced IL-1β secretion, whereas ATP-induced NLRP3 inflammasome activation, which does not require endocytic routes to activate the NLRP3 inflammasome [12] , [22] , was largely unaffected ( Fig. 2a ). These data suggest that the cellular internalization of liposomes is an essential step for liposome-induced NLRP3 inflammasome activation. 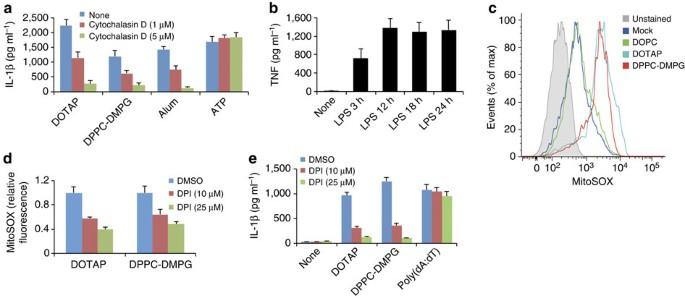Figure 2: Liposome-induced inflammasome activation requires uptake of liposomes and ROS. (a) IL-1β from the supernatants of PMA-primed THP1 cells that were pretreated with cytochalasin D before stimulation with indicated liposomes (DOTAP liposome 40 μg ml−1, DPPC-DMPG liposomes 100 μg ml−1), alum (500 μg ml−1) or ATP (2 mM). (b) ELISA for TNF from the supernatants of wild-type BMDMs that were stimulated with 100 ng ml−1LPS for various periods of time as indicated. (c) Mitochondrial ROS production was measured by flow cytometry in LPS-primed BMDMs that were stimulated with indicated liposomes (30 μg ml−1) and labelled with MitoSOX. (d) LPS-primed wild-type BMDMs were pretreated with DPI for 30 min and then stimulated with indicated liposomes (30 μg ml−1) for 6 h. The cells were then stained with MitoSOX and the levels of mitochondrial ROS were normalized to the untreated controls (n=3). (e) ELISA for IL-1β from the supernatants of LPS-primed (18 h) BMDMs that were pretreated with DPI before stimulation with indicated liposomes (30 μg ml−1) or poly(dA:dT) (2 μg ml−1). The data in (a,b,d,e) are shown as mean±s.d., and the data are representative of three (a,b,d,e) and four (c) independent experiments. Figure 2: Liposome-induced inflammasome activation requires uptake of liposomes and ROS. ( a ) IL-1β from the supernatants of PMA-primed THP1 cells that were pretreated with cytochalasin D before stimulation with indicated liposomes (DOTAP liposome 40 μg ml −1 , DPPC-DMPG liposomes 100 μg ml −1 ), alum (500 μg ml −1 ) or ATP (2 mM). ( b ) ELISA for TNF from the supernatants of wild-type BMDMs that were stimulated with 100 ng ml −1 LPS for various periods of time as indicated. ( c ) Mitochondrial ROS production was measured by flow cytometry in LPS-primed BMDMs that were stimulated with indicated liposomes (30 μg ml −1 ) and labelled with MitoSOX. ( d ) LPS-primed wild-type BMDMs were pretreated with DPI for 30 min and then stimulated with indicated liposomes (30 μg ml −1 ) for 6 h. The cells were then stained with MitoSOX and the levels of mitochondrial ROS were normalized to the untreated controls ( n =3). ( e ) ELISA for IL-1β from the supernatants of LPS-primed (18 h) BMDMs that were pretreated with DPI before stimulation with indicated liposomes (30 μg ml −1 ) or poly(dA:dT) (2 μg ml −1 ). The data in ( a , b , d , e ) are shown as mean±s.d., and the data are representative of three ( a , b , d , e ) and four ( c ) independent experiments. Full size image We also sought to determine whether the lysosome-cathepsin B pathway was involved in liposome-induced NLRP3 inflammasome activation. First, we found that the pharmacological inhibition of lysosomal acidification, a process critical for crystal-induced inflammasome activation [12] , did not significantly affect liposome-induced NLRP3 inflammasome-mediated IL-1β secretion ( Supplementary Fig. S7a ). Furthermore, we also observed that lysosomal cathepsin B was not necessary for liposome-triggered NLRP3 inflammasome activation because cathepsin B-deficient macrophages had only a minimal reduction in the amount of secreted IL-1β after liposome stimulation ( Supplementary Fig. S7b ). Notably, we observed that liposome-induced IL-1β secretion was decreased in BMDMs that were pretreated with a cathepsin B inhibitor, CA-074-Me ( Supplementary Fig.S7c ). These seemingly conflicting data may be due to the potential off-target side effects of CA-074-Me [12] , [27] , [28] . Taken together, these data indicate that liposomes may either activate the NLRP3 inflammasome in a lysosome-independent manner or that several lysosomal cathepsins, such as cathepsins B and L, are functionally redundant in mediating liposome-induced NLRP3 inflammasome activation. Liposomes induce mitochondrial ROS to activate inflammasome Although mitochondrial ROS are essential for activation of the NLRP3 inflammasome [17] , [18] , [19] , [20] , a recent study also suggested a role for ROS during the first priming step of pro-IL-1β synthesis [29] . Therefore, to specifically investigate the role of ROS during activation of the NLRP3 inflammasome activation but not during pro-IL-1β synthesis, we added ROS inhibitors after the synthesis of pro-IL-1β was completed. This was achieved through prolonged LPS stimulation to saturate NF-κB activation before ROS inhibition. As shown in Fig. 2b , prolonged LPS priming for 18 h maximized the level of NF-κB-mediated transcription, which was measured by the production of NF-κB-dependent TNF. We then evaluated whether different liposomes could induce mitochondrial ROS production. Notably, only the charged liposomes, but not neutral liposomes, induced the robust generation of mitochondrial ROS in LPS-primed macrophages ( Fig. 2c ). Moreover, even in the absence of an LPS-priming step, charged liposomes remained capable of increasing the mitochondrial ROS levels, suggesting that LPS pre-stimulation is not necessary for mitochondrial ROS induction ( Supplementary Fig. S8 ). Next, we used the pharmacological inhibitor diphenyleneiodonium (DPI), which blocks mitochondrial ROS production when used at high concentrations [30] , [31] , to further investigate whether mitochondrial ROS were involved in liposome-induced NLRP3 inflammsome activation. The addition of DPI before liposome stimulation drastically reduced liposome-induced mitochondrial ROS production and IL-1β release ( Fig. 2d ). Notably, the reduction in IL-1β secretion was not owing to the inhibition of NF-κB activation by DPI because neither the levels of pro-IL-1β or Nlrp3 were significantly changed after the 18-h LPS-priming step ( Supplementary Fig. S9 ). In contrast to DPI, pretreatment of the macrophage with VAS2870, which blocks NADPH oxidase (NOX)-generated ROS [32] , did not affect liposome-induced IL-1β secretion, suggesting that mitochondria, rather than NOX-derived ROS, drive the NLRP3 inflammasome activation ( Supplementary Fig. S10 ). Moreover, because activation of the AIM2 inflammasome by poly(dA:dT) was not affected by DPI treatment ( Fig. 2e ), the inhibition of mitochondrial ROS seemed to specifically affect the NLRP3 inflammasome. Similar results were also observed when other ROS inhibitors, such as (2R, 4R)-4-aminopyrrolidine-2,4-dicarboxylate (APDC) or N -acetyl-cysteine (NAC), were used (data not shown). Taken together, these data indicate that mitochondrial ROS production is essential for NLRP3 inflammasome activation by charged liposomes and that the failure of neutral liposomes to activate the NLRP3 inflammasome directly correlates with their inability to induce mitochondrial ROS. Particulates induce a ROS-dependent Ca 2+ influx via TRPM2 Our findings indicated that, similar to crystals [33] , liposomes activate the NLRP3 inflammasome via the induction of mitochondrial ROS. However, little is known about the mechanism by which ROS promote NLRP3 inflammasome activation. Owing to the existence of a diverse pool of stimuli [21] , these agonists may activate a common signalling intermediate that directs assembly of the NLRP3 inflammasome. Recently, it has been shown that accumulation of ROS can induce a calcium influx via the TRPM2 channel [34] , [35] . TRPM2 is expressed by immune cells, such as dendritic cells, monocytes, macrophages, PMNs and lymphocytes, and is a calcium-permeable non-selective cation channel that has a crucial role in innate immune regulation [36] . TRPM2-mediated calcium influx has been implicated in ROS-induced chemokine production in monocytes [34] . Notably, TRPM2-deficient mice are also susceptible to infection of Listeria monocytogenes [37] , a known activator of the NLRP3 inflammasome [22] , [38] . As calcium appears to be a key mediator of various signalling events under stressed conditions, we hypothesize that liposomes/crystals induce ROS-dependent TRPM2-mediated calcium influx, which eventually signals assembly and activation of the NLRP3 inflammasome. As shown in Fig. 3a , we first observed that charged liposomes or crystals induced the increase in the concentration of intracellular free calcium ([Ca 2+ ] i ). This elevation in [Ca 2+ ] i was owing to calcium influx across the plasma membrane because the removal of extracellular calcium from the buffer solution dramatically inhibited the increase of [Ca 2+ ] i ( Fig. 3c and Supplementary Fig. S11 ). Furthermore, blockade of mitochondrial ROS by DPI also prevented liposome-/crystal-induced calcium influx, suggesting that calcium influx is ROS-dependent. Notably, BMDMs deficient in TRPM2 had similar defects in calcium influx after liposome/crystal stimulation, indicating that calcium influx is mediated by the TRPM2 channel ( Fig. 3c and Supplementary Fig. S11 ). To further verify the role of TRPM2 in mediating calcium influx, we tested whether inhibition of TRPM2 activation affected liposome-/crystal-induced calcium influx. TRPM2 channel can be gated by ADP-ribose, a metabolic product formed during cellular exposure to ROS [36] , [37] . Therefore, we treated LPS-primed wild-type BMDMs with DPQ, an inhibitor of poly(ADP-ribose) polymerase, to prevent ADP-ribose accumulation [39] , [40] before the addition of liposomes/crystals to determine whether the calcium influx was affected. As expected, DPQ significantly reduced calcium influx in response to stimulation with particles ( Fig. 3c and Supplementary Fig. S11 ). These data collectively indicate that stimulation of macrophages with either liposomes or crystals can trigger ROS-dependent TRPM2-mediated calcium influx. 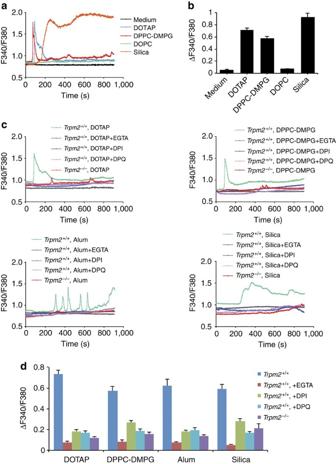Figure 3: Liposomes and crystals induce ROS-dependent Ca2+influx via the TRPM2 channel. (a) The change in [Ca2+]iover time was represented by the fluorescence of Fura-2 at 340 nm to that at 380 nm (F340/F380) and (b) the maximum [Ca2+]ielevations, represented by ΔF340/F380, are shown in LPS-primed wild-type BMDMs treated with medium alone, cationic liposomes (DOTAP, 30 μg ml−1), neutral liposomes (DOPC, 30 μg ml−1), anionic liposomes (DPPC-DMPG, 30 μg ml−1) or silica crystals (300 μg ml−1). (c) The time-dependent change in [Ca2+]i, represented by F340/F380, in the LPS-primedTrpm2+/+BMDMs cultured in calcium-containing solution that were pretreated with DPI (25 μM) or DPQ (200 μM) for 45 min before the addition of the indicated liposomes (30 μg ml−1) or crystals (alum, 400 μg ml−1; silica, 300 μg ml−1) is shown. The same doses of liposomes or crystals were also used to stimulate the LPS-primedTrpm2−/−BMDMs cultured in calcium-containing solution. The [Ca2+]ichange over time, represented by F340/F380, after stimulation with liposomes or crystals in LPS-primedTrpm2+/+BMDMs cultured in calcium-free 0.5 mM EGTA-containing solution is also shown. Inflammasome agonists were added 1 min after the initiation of calcium recording as shown in (a,c). (d) The maximum [Ca2+]ielevations, represented by ΔF340/F380, are shown for LPS-primed BMDMs in response to the stimulations described in (c). The data are representative of at least three independent experiments and are shown as mean±s.e.m. in (b,d) (n=22–31 in (b), andn=21–34 in (d)). Figure 3: Liposomes and crystals induce ROS-dependent Ca 2+ influx via the TRPM2 channel. ( a ) The change in [Ca 2+ ] i over time was represented by the fluorescence of Fura-2 at 340 nm to that at 380 nm (F340/F380) and ( b ) the maximum [Ca 2+ ] i elevations, represented by ΔF340/F380, are shown in LPS-primed wild-type BMDMs treated with medium alone, cationic liposomes (DOTAP, 30 μg ml −1 ), neutral liposomes (DOPC, 30 μg ml −1 ), anionic liposomes (DPPC-DMPG, 30 μg ml −1 ) or silica crystals (300 μg ml −1 ). ( c ) The time-dependent change in [Ca 2+ ] i , represented by F340/F380, in the LPS-primed Trpm2 +/+ BMDMs cultured in calcium-containing solution that were pretreated with DPI (25 μM) or DPQ (200 μM) for 45 min before the addition of the indicated liposomes (30 μg ml −1 ) or crystals (alum, 400 μg ml −1 ; silica, 300 μg ml −1 ) is shown. The same doses of liposomes or crystals were also used to stimulate the LPS-primed Trpm2 −/− BMDMs cultured in calcium-containing solution. The [Ca 2+ ] i change over time, represented by F340/F380, after stimulation with liposomes or crystals in LPS-primed Trpm2 +/+ BMDMs cultured in calcium-free 0.5 mM EGTA-containing solution is also shown. Inflammasome agonists were added 1 min after the initiation of calcium recording as shown in ( a , c ). ( d ) The maximum [Ca 2+ ] i elevations, represented by ΔF340/F380, are shown for LPS-primed BMDMs in response to the stimulations described in ( c ). The data are representative of at least three independent experiments and are shown as mean±s.e.m. in ( b , d ) ( n =22–31 in ( b ), and n =21–34 in ( d )). Full size image Ca 2+ influx via TRPM2 directs particle-induced IL-1β release We next determined whether TRPM2-mediated calcium influx was critical for IL-1β release. Trpm2 −/− BMDMs demonstrated significantly reduced IL-1β secretion in responses to stimulation with the liposomes DOTAP and DPPC-DMPG or the crystals of alum, silica and MSU. In contrast, poly(dA:dT)-induced IL-1β secretion, which is AIM2 inflammasome-dependent [24] , [25] , was largely unaffected ( Fig. 4a ). Similarly, the removal of extracellular calcium from the culture medium significantly impaired the particulate agonist-, but not poly(dA:dT)-, induced IL-1β release ( Fig. 4a ). 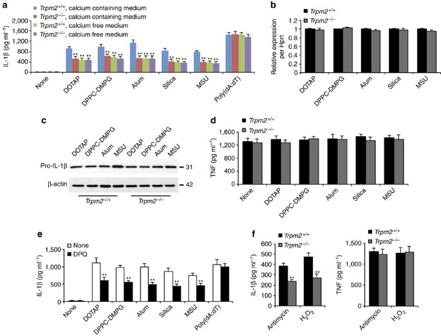Figure 4: Ca2+influx via TRPM2 is crucial for liposome- or crystal-induced IL-1β secretion. ELISA for IL-1β (a) or TNF (d) from the supernatants of LPS-primed wild-type (Trpm2+/+) orTrpm2−/−BMDMs that were stimulated with indicated liposomes (30 μg ml−1), crystals (alum, 250 μg ml−1; silica and MSU crystals, 200 μg ml−1) or poly(dA:dT) (2 μg ml−1) for 6 h in calcium-containing or calcium-free medium. (b) The levels of pro-IL-1β mRNA were quantified by real-time RT-PCR in LPS-primedTrpm2+/+orTrpm2−/−BMDMs after stimulation with indicated liposomes and crystals as in (a). The gene expression data are presented as expression relative to HPRT1, and the relative gene expression levels in wild-type macrophages were designated as 1. (c) Immunoblots for pro-IL-1β and β-actin in the cell lysates from LPS-primedTrpm2+/+orTrpm2−/−BMDMs after stimulation with liposomes or crystals as in (a). (e) IL-1β from the supernatants of LPS-primed wild-type BMDMs that were pretreated with DPQ (200 μM) followed by inflammasome agonist stimulation as ina. (f) IL-1β (left) or TNF (right) from the supernatants of LPS-primed wild-type BMDMs that were stimulated with antimycin A (20 μg ml−1) or H2O2(10 mM) for 6 h. Experiments described in (b–f) were performed in calcium-containing medium. All data are representative of at least three independent experiments, and are shown as mean±s.d. in (a,b,d–f). *P<0.05 and **P<0.01 versus controls. Statistical significance was determined by the standard two-tailed Student’st-test. Figure 4: Ca 2+ influx via TRPM2 is crucial for liposome- or crystal-induced IL-1β secretion. ELISA for IL-1β ( a ) or TNF ( d ) from the supernatants of LPS-primed wild-type ( Trpm2 +/+ ) or Trpm2 −/− BMDMs that were stimulated with indicated liposomes (30 μg ml −1 ), crystals (alum, 250 μg ml −1 ; silica and MSU crystals, 200 μg ml −1 ) or poly(dA:dT) (2 μg ml −1 ) for 6 h in calcium-containing or calcium-free medium. ( b ) The levels of pro-IL-1β mRNA were quantified by real-time RT-PCR in LPS-primed Trpm2 +/+ or Trpm2 −/− BMDMs after stimulation with indicated liposomes and crystals as in ( a ). The gene expression data are presented as expression relative to HPRT1, and the relative gene expression levels in wild-type macrophages were designated as 1. ( c ) Immunoblots for pro-IL-1β and β-actin in the cell lysates from LPS-primed Trpm2 +/+ or Trpm2 −/− BMDMs after stimulation with liposomes or crystals as in ( a ). ( e ) IL-1β from the supernatants of LPS-primed wild-type BMDMs that were pretreated with DPQ (200 μM) followed by inflammasome agonist stimulation as in a . ( f ) IL-1β (left) or TNF (right) from the supernatants of LPS-primed wild-type BMDMs that were stimulated with antimycin A (20 μg ml −1 ) or H 2 O 2 (10 mM) for 6 h. Experiments described in ( b – f ) were performed in calcium-containing medium. All data are representative of at least three independent experiments, and are shown as mean±s.d. in ( a , b , d – f ). * P <0.05 and ** P <0.01 versus controls. Statistical significance was determined by the standard two-tailed Student’s t -test. Full size image Furthermore, we observed that the decrease in the mature IL-1β secretion in Trpm2 −/− BMDMs was not owing to the reduction in either pro-IL-1β or NLRP3 levels, the genes for which are regulated by NF-κB [21] , [41] because TRPM2 deficiency affected neither pro-IL-1β nor NLRP3 ( Fig. 4b and data not shown). Consistent with this finding, TNF secretion was not affected by TRPM2 deficiency ( Fig. 4d ). Moreover, the inhibition of TRPM2 activation by DPQ also significantly impaired liposome-/crystal-, but not poly(dA:dT)-, induced IL-1β secretion ( Fig. 4e ). In contrast to the wild-type cells, Trpm2 −/− BMDMs did not display any further reduction in IL-1β secretion after DPQ treatment ( Supplementary Fig. S12 ), indicating that DPQ treatment specifically blocked TRPM2-mediated IL-1β release. It has been shown that the inhibition of key enzymes in the mitochondrial respiratory chain can artificially increase the levels of mitochondrial ROS and trigger spontaneous NLRP3 inflammasome activation in the absence of inflammasome stimuli [20] , therefore we next verified the role of TRPM2 in mediating IL-1β release under these conditions. To do so, we artificially induced the accumulation of mitochondrial ROS with antimycin A, an inhibitor that specifically blocks the respiratory chain complex III, and determined whether TRPM2 deficiency affected antimycin A-induced IL-1β release. Indeed, we found that Trpm2 −/− BMDMs had significantly reduced secretion of IL-1β, but not TNF ( Fig. 4f ). Consistently, TRPM2 deficiency also decreased IL-1β secretion in response to direct stimulation with ROS, such as H 2 O 2 ( Fig. 4f ). Together, these results suggest a critical role for TRPM2-mediated calcium influx in bioactive IL-1β release, and demonstrate that TRPM2 deficiency specifically impairs the processing of immature pro-IL-1β into its mature form. It should be noted that in addition to TRPM2-dependent IL-1β release, liposomes/crystals also induced TRPM2-independent IL-1β secretion. This effect was most likely mediated by endoplasmic reticulum (ER)-calcium release via IP 3 R, as suggested in a recent study by Murakami et al . [15] In support of the hypothesis that calcium influx and ER calcium release are both essential for NLRP3 inflammasome activation, we observed that the intracellular calcium chelator BAPTA-AM, which blocks [Ca 2+ ] i elevation regardless of the source of calcium, almost completely inhibited IL-1β release ( Supplementary Fig. S13 ) whereas the inhibition of either calcium influx ( Fig. 4a ) or intracellular ER calcium release [15] only partially reduced IL-1β secretion. Together, these results demonstrate that both calcium influx and ER calcium release are critical for activation of the NLRP3 inflammasome. TRPM2 deficiency inhibits caspase-1 activation To determine the mechanism by which TRPM2 deficiency leads to impaired processing of bioactive IL-1β, we tested whether Trpm2 −/− BMDMs were defective in caspase-1 activation. As shown in Fig. 5a , deficiency in TRPM2 or the blockade of [Ca 2+ ] i increase via BAPTA-AM that drastically reduced the level of mature caspase-1 in response to liposomes or crystals. This defect was not owing to impaired mitochondrial ROS production because neither genetic ablation of TRPM2 nor removal of extracellular calcium impaired mitochondrial ROS production after liposome stimulation ( Fig. 5c–e , and Supplementary Fig. S14 ). Moreover, we found that Nlrp3 −/− macrophages displayed a comparable level of calcium influx as wild-type cells in response to liposome stimulation ( Fig. 5f ), suggesting that TRPM2-mediated calcium influx is an early event before assembly of the NLRP3 inflammasome. Together, these data indicate that ROS-dependent calcium influx via the TRPM2 channel is critical for NLRP3 inflammasome-mediated caspase-1 activation. 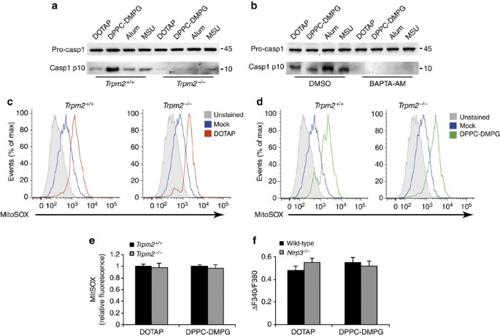Figure 5: TRPM2 directs caspase-1 activation but is dispensable for mitochondrial ROS production. (a) Immunoblots of procaspase-1 in lysates and caspase-1 p10 in culture supernatants of LPS-primedTrpm2+/+andTrpm2−/−BMDMs that were stimulated with indicated liposomes (30 μg ml−1) or crystals (250 μg ml−1). (b) Immunoblots of procaspase-1 and caspase-1 p10 in LPS-primed wild-type BMDMs that were preteated with either BAPTA-AM (25 μM) or DMSO before stimulation with the indicated liposomes (50 μg ml−1) and crystals (400 μg ml−1). One of three independent experiments is shown in (a,b). (c–e) LPS-primedTrpm2+/+orTrpm2−/−BMDMs were treated with indicated liposomes (30 μg ml−1) for 6 h. The cells were then stained with MitoSOX and the levels of mitochondrial ROS were measured by flow cytometry (c,d). The data are representative for three experiments and are normalized to the untreated controls (e,n=3). (f) The maximum [Ca2+]ielevations, represented by ΔF340/F380, are shown for LPS-primed immortalized murine wild-type orNlrp3−/−macrophages in response to stimulation with liposomes (70 μg ml−1). The data are shown as mean±s.e.m. (n=23–28), and are representative of two independent experiments. Figure 5: TRPM2 directs caspase-1 activation but is dispensable for mitochondrial ROS production. ( a ) Immunoblots of procaspase-1 in lysates and caspase-1 p10 in culture supernatants of LPS-primed Trpm2 +/+ and Trpm2 −/− BMDMs that were stimulated with indicated liposomes (30 μg ml −1 ) or crystals (250 μg ml −1 ). ( b ) Immunoblots of procaspase-1 and caspase-1 p10 in LPS-primed wild-type BMDMs that were preteated with either BAPTA-AM (25 μM) or DMSO before stimulation with the indicated liposomes (50 μg ml −1 ) and crystals (400 μg ml −1 ). One of three independent experiments is shown in ( a , b ). ( c – e ) LPS-primed Trpm2 +/+ or Trpm2 −/− BMDMs were treated with indicated liposomes (30 μg ml −1 ) for 6 h. The cells were then stained with MitoSOX and the levels of mitochondrial ROS were measured by flow cytometry ( c , d ). The data are representative for three experiments and are normalized to the untreated controls ( e , n =3). ( f ) The maximum [Ca 2+ ] i elevations, represented by ΔF340/F380, are shown for LPS-primed immortalized murine wild-type or Nlrp3 −/− macrophages in response to stimulation with liposomes (70 μg ml −1 ). The data are shown as mean±s.e.m. ( n =23–28), and are representative of two independent experiments. Full size image Along with the role of calcium influx in activation of the NLRP3 inflammasome, potassium efflux has been shown to be essential for inflammasome activation by most, if not all, NLRP3 inflammasome agonists [14] , [33] . It appears that the mobilization of both cations across the plasma membrane is crucial for NLRP3 inflammasome activation. Consistent with a recent study [42] , we found that the blockade of potassium efflux did not prevent calcium influx induced by NLRP3 inflammasome agonists ( Supplementary Fig. S15 ), which further verifies that in addition to potassium efflux, calcium influx is also a crucial event for NLRP3 inflammasome activation. As TRPM2 is a non-selective cation channel that allows the passage of both calcium and potassium [36] , it is possible that TRPM2 deficiency may also affect potassium efflux. However, as the removal of extracellular calcium did not further decrease the particulate-induced NLRP3 inflammasome activation in Trpm2 −/− BMDMs ( Fig. 4a ), the defect of NLRP3 inflammasome activation in TRPM2-deficient cells is most likely owing to impaired calcium influx. It should be noted that ATP-induced NLRP3 inflammasome activation was also primarily dependent on calcium influx ( Supplementary Fig. S16 ). However, in contrast to particulate agonists of the NLRP3 inflammasome, ATP uses P2X 7 , but not TRPM2, to induce calcium influx and NLRP3 inflammasome activation ( Supplementary Fig. S16 ). Consistent with this notion, deficiency in P2X 7 did not affect calcium influx triggered by particulate stimuli ( Supplementary Fig. S17 ). Taken together, these results suggest that calcium influx is a general proximal step during NLRP3 inflammasome activation, and that different activators of the NLRP3 inflammasome may use distinct plasma membrane ion channels to mediate calcium influx. TRPM2 is crucial for NLRP3 inflammasome activation in vivo To further validate the role of TRPM2 in mediating NLRP3 inflammasome activation in vivo , we determined whether TRPM2 deficiency affected crystal-/liposome-induced IL-1β secretion and subsequent neutrophil recruitment after intraperitoneal injections of these particulate stimuli. We first observed that the level of IL-1β in the peritoneal fluid of the Trpm2 −/− mice was significantly reduced as compared with that from wild-type mice after injection with either MSU crystals or DOTAP liposomes ( Fig. 6a ). Moreover, particle-induced neutrophil recruitment was also significantly decreased in Trpm2 −/− mice, which was similar to that observed in Il1r1 −/− mice ( Fig. 6b ). In contrast, neutrophil recruitment was not affected by either TRPM2 or IL-1R deficiency in response to an intraperitoneal challenge with zymosan, a Toll-like receptor 2 agonist ( Supplementary Fig.S18 ). These data collectively indicate that TRPM2 is essential for NLRP3 inflammasome activation in vivo . 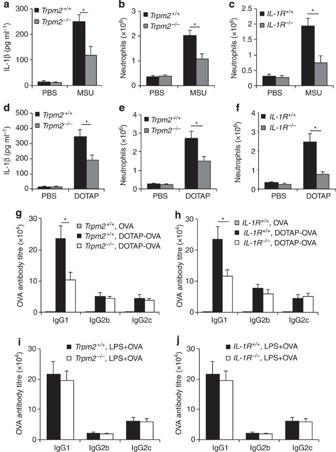Figure 6: TRPM2 is critical for particle-induced IL-1β release and subsequent immune responsesin vivo. The IL-1β concentration (a,d) and neutrophil recruitment (b,c,e,f) were quantified in peritoneal lavage fluid from wild-type (Il1r1+/+andTrpm2+/+),Il1r1−/−orTrpm2−/−mice 6 h after intraperitoneal injection of PBS supplemented with either MSU crystals (a–c) or DOTAP liposomes (d–f). The data are representative of two independent experiments (mean and s.e.m. of three to five mice per group). (g–j) Six- to eight-week old female wild-type (Trpm2+/+andIl1r1+/+),Trpm2−/−(g,i)or Il1r1−/−(h,j) mice were subcutaneously immunized on day 0 and day 14 with 40 μg per mouse OVA alone or the same amount of OVA encapsulated within DOTAP liposomes (g,h) or mixed with LPS (25 μg per mouse,i,j). On day 24, the mice were killed, and sera were collected and analysed for OVA-specific IgG1, IgG2b and IgG2c levels by ELISA. The data are shown as geometrical mean±s.e.m., and are representative of at least two independent experiments (n=4–5 mice per group). *P<0.05 versus controls. Statistical significance was determined by the standard two-tailed Student’st-test. Figure 6: TRPM2 is critical for particle-induced IL-1β release and subsequent immune responses in vivo . The IL-1β concentration ( a , d ) and neutrophil recruitment ( b , c , e , f ) were quantified in peritoneal lavage fluid from wild-type ( Il1r1 +/+ and Trpm2 +/+ ), Il1r1 −/− or Trpm2 −/− mice 6 h after intraperitoneal injection of PBS supplemented with either MSU crystals ( a – c ) or DOTAP liposomes ( d – f ). The data are representative of two independent experiments (mean and s.e.m. of three to five mice per group). ( g – j ) Six- to eight-week old female wild-type ( Trpm2 +/+ and Il1r1 +/+ ), Trpm2 −/− ( g , i ) or Il1r1 −/− ( h , j ) mice were subcutaneously immunized on day 0 and day 14 with 40 μg per mouse OVA alone or the same amount of OVA encapsulated within DOTAP liposomes ( g , h ) or mixed with LPS (25 μg per mouse, i , j ). On day 24, the mice were killed, and sera were collected and analysed for OVA-specific IgG1, IgG2b and IgG2c levels by ELISA. The data are shown as geometrical mean±s.e.m., and are representative of at least two independent experiments ( n =4–5 mice per group). * P <0.05 versus controls. Statistical significance was determined by the standard two-tailed Student’s t -test. Full size image Finally, we tested whether deficiency in TRPM2, which results in decreased IL-1β secretion, would affect the adjuvanticity of liposomes in vivo . As shown in Fig. 6g , the level of ovalbumin (OVA)-specific IgG1 was significantly reduced in Trpm2 −/− mice after immunization with OVA-encapsulated DOTAP liposomes. Furthermore, because a role for the IL-1β-IL-1 receptor signalling axis in mediating Th2 responses has been previously suggested [43] , we further tested whether the inhibition of IL-1 receptor signalling influenced the levels of antigen-specific antibodies after immunization with antigen-encapsulated liposomes. Similar to Trpm2 −/− mice, Il1r1 −/− mice also demonstrated a significant reduction in OVA-specific IgG1 levels compared with the wild-type mice ( Fig. 6h ). However, in contrast to the liposomal adjuvant, a deficiency in either TRPM2 or IL-1R did not impair the optimal levels of anti-OVA antibodies when LPS, a Toll-like receptor 4 agonist, was used as the adjuvant ( Fig. 6i ), which suggests that TRPM2- and IL-1R-deficient mice do not have a general defect in mounting an antibody response. Taken together, these data indicate that TRPM2 and IL-1R are essential for the induction of an optimal antibody response against the antigens that are encapsulated within liposomes. Liposomes are promising immune adjuvants and delivery vectors for the treatment of both infectious and cancerous diseases [1] , [3] , [4] . Therefore, understanding the innate immune recognition process for liposomes will not only mechanistically define/improve their adjuvant effect but also help to prevent any undesirable inflammatory responses, particularly when liposomes are used as drug-delivery vehicles for anti-cancer therapies. In this study, we identified the NLRP3 inflammasome as a novel innate immune sensor for liposomes. Notably, only the charged, but not neutral, liposomes activated the NLRP3 inflammasome, which is most likely owing to the fundamental differences in their induction of mitochondrial ROS. As the plasma membrane potential is tightly associated with the oxidative state in phagocytes [44] , [45] , [46] , it is plausible that charged, but not neutral, liposomes could induce cellular oxidative stress via alteration of the plasma membrane potential, which would eventually result in NLRP3 inflammasome activation. Therefore, charged liposomes may be more suitable as immune adjuvants, whereas neutral liposomes may be more suitable as delivery vectors for anti-cancer drugs. Although an essential role for mitochondrial ROS has recently been implicated in activation of the NLRP3 inflammasome [17] , [18] , the precise mechanism underlying ROS-induced inflammasome activation remains elusive. In this study, we identified a novel signalling axis originating from ROS production, followed by TRPM2-mediated calcium influx and ultimately activation of the NLRP3 inflammasome. Therefore, our results provide at least one mechanistic link that connects oxidative stress with NLRP3 inflammasome activation. In addition to TRPM2-dependent IL-1β release, we observed that a portion of particle-induced IL-1β secretion was independent of TRPM2-mediated calcium influx but instead was dependent on calcium release from intracellular stores. This observation is consistent with a recent report by Murakami et al . [15] that demonstrated a role for IP 3 R-mediated calcium release from the ER in the activation of the NLRP3 inflammasome. Although it is clear that both calcium influx and ER calcium release are critical for IL-1β secretion, how multiple calcium mobilization events cooperatively trigger NLRP3 inflammasome activation remains to be further defined. Recently, a report by Zhou et al . [20] demonstrated a close interaction between the ER and mitochondria in response to NLRP3 inflammasome stimuli. As calcium overload in mitochondria is essential for ROS production, it is plausible that ER-mitochondria contact may be beneficial for rapid calcium flow from the ER into mitochondria, which may facilitate the generation of sufficient mitochondrial ROS, particularly at later stage during activation of the NLRP3 inflammasome. Moreover, Murakami et al . [15] have also demonstrated that in addition to facilitating mitochondrial ROS production, ER-derived calcium is also essential for mitochondria to maintain a damaged state. Mitochondrial damage has been shown to induce the release of mitochondrial DNA into the cytosol, which also activates the inflammasomes [19] , [47] . In addition to mitochondrial DNA, our study demonstrates that ROS released from the damaged mitochondria activate the TRPM2 channel, which results in calcium influx across the plasma membrane. As blocking TRPM2-mediated calcium mobilization drastically impaired caspase-1 activation and did not affect mitochondrial ROS production, it is possible that, unlike ER-derived calcium, TRPM2-mediated calcium influx may directly signal activation of the NLRP3 inflammasome. Based on our current study and a previous report by Murakami et al . [15] , it appears that calcium mobilization is a critical step during NLRP3 inflammasome activation. Calcium is a key signalling mediator for a number of cellular proteases, protein kinases and phospholipases, some of which may be involved in NLRP3 inflammasome activation. Consistent with this notion, ERK1/2 kinase has been implicated in regulating activation of the NLRP3 inflammasome [48] . Similarly, we have preliminary data indicating that the inhibition of protein kinase C α also partially impairs NLRP3 inflammasome activation (unpublished results). These calcium-dependent enzymes may function to either proteolytically inactivate a negative regulator or activate a positive regulator of NLRP3, resulting in the assembly of the inflammasome complex. Finally, accumulating evidence has suggested that dysregulation of the NLRP3 inflammasome is tightly associated with many inflammatory disorders, such as gout, atherosclerosis, silicosis, asbestosis and Alzheimer’s disease [49] , [50] . In this study, we demonstrated that TRPM2 deficiency drastically impairs the inflammatory response induced by MSU crystals, the casual agent of gout. This finding has therefore suggested a therapeutic potential of targeting TRPM2 to treat NLRP3 inflammasome-associated autoinflammatory diseases. Furthermore, other studies have also linked the NLRP3 inflammasome to a number of metabolic diseases, including obesity and type 2 diabetes [51] , [52] , [53] . For instance, NLRP3 deficiency protects mice from high-fat diet-induced obesity, and the saturated fatty acid palmitate, which is found in high-fat diets, can induce NLRP3 inflammasome-mediated IL-1β secretion, which interferes with insulin signalling and eventually results in reduced glucose tolerance and insulin sensitivity. As our results indicate a role for TRPM2 in NLRP3 inflammasome activation, blocking TRPM2 would be expected to rescue metabolic disorders that are a result of a high-fat diet. In support of this hypothesis, a recent study suggested that TRPM2-deficient mice have attenuated obesity-mediated inflammation, and that TRPM2 deletion can protect mice from developing diet-induced obesity and insulin resistance [54] . Together, these studies highlight the therapeutic potential of targeting TRPM2 to treat autoinflammatory and metabolic disorders associated with undesirable activation of the NLRP3 inflammasome. Mice C57BL/6, Il1r1 −/− and P2X 7 −/− mice were purchased from Jackson Laboratories. Trpm2 −/− mice were a generous gift from Dr Yasuo Mori and have been previously described [34] . Trpm2 −/− mice were backcrossed with C57BL/6 mice for at least five generations before use in the experiments described. Trpm 2 −/− mice and their wild-type littermates ( Trpm2 +/+ ) were used in these studies. All mice were bred and maintained in the animal facility at Loyola University Chicago and were treated in accordance with the guidelines of the Institutional Animal Care and Use Committee of Loyola University Chicago. Reagents 1,2-Dioleoyl-3-trimethylammonium-propane (DOTAP), 3β-(N-(N′,N′-dimethylaminoethane)-carbamoyl)cholesterol hydrochloride (DC-Chol), dimethyldioctadecylammonium (bromide salt) (DDA), 1,2-dioleoyl-sn-glycero-3-phosphocholine (DOPC), 1,2-dipalmitoyl-sn-glycero-3-phosphocholine (DPPC), 1,2-dimyristoyl-sn-glycero-3-phospho-(1′-rac-glycerol) (DMPG) and L-α-phosphatidylcholine (soy extract) were purchased from Avanti Polar Lipids (Alabaster, AL). Track-etch polycarbonate membranes (2 μm, 800 nm, 400 nm, 200 nm and 100 nm) were from Millipore. The Lipex liposomes extruder was from Northern Lipids and other common lab chemicals and reagents were from Sigma-Aldrich and Fisher Scientific. Cholesterol, ovalbumin, silica, ATP, PMA, cytochalasin D, uricase, bafilomycin A1, Ca-074-Me, H 2 O 2 , antimycin and BAPTA-AM were from Sigma-Aldrich. Ultrapure LPS, zymosan, and poly(dA:dT), and glibenclamide were from Invivogen. zYVAD-fmk, APDC and DPQ were from Alexis Biochemicals. DPI was from Calbiochem. Monosodium urate crystals, VAS2870 and NAC were from Enzo Lifescience. Imject Alum and streptavidin-HRP were from Pierce. Lipofectamine 2000, MitoSOX and fura-2-AM were from Invitrogen. Calcium-free and calcium-containing DMEM media were from US Biologicals. The lactate dehydrogenase (LDH) assay kit was from Roche. Antibodies used for immunoblotting were as follows: anti-mouse caspase-1 (sc-514, Santa Cruz Biotechnology), anti-mouse β-actin (sc-1615 HRP, Santa Cruz Biotechnology) and anti-mouse IL-1β (AF-401-NA, R&D Systems). Antibodies used for determining OVA-specific IgG isotypes IgG1 and IgG2b were from Biolegend, and the antibody for mouse IgG2c was from Bethyl Laboratories. Liposomes formulations A total of 16 different liposomes formulations (see Supplementary Information ) were produced by Encapsula NanoSciences. The liposomes were made using the dehydration–rehydration method. The lipids were dissolved in chloroform in a round bottom flask, and the solvent in the flask was then evaporated using a Büchi (RE-121) rotary evaporator (Flawil, Switzerland) under a vacuum for 4 h, resulting in the formation of a thin lipid film. The thin lipid film was hydrated with deionized water for 2 h at 37 °C and then over night at 4 °C. The milky solution of liposomes was extruded 25 times through an appropriately sized polycarbonate membrane filter using a Lipex extruder connected to a high-pressure nitrogen cylinder to produce liposomes of the desired sizes. For example, liposomes were passed through a 100-nm polycarbonate membrane filter 25 times to produce 100-nm liposomes. To formulate OVA-encapsulated liposomes, the thin lipid film was hydrated with a solution of OVA in deionized water. The liposomes were sized to 400 nm. The non-encapsulated OVA was separated using 100 K dialysis membrane tubing (Spectrum Laboratories). The amount of the encapsulated OVA was determined by BCA assay using a BCA protein assay kit (ThermoFisher Scientific). Cell culture and stimulation Human THP-1 cells (ATCC) were grown in RPMI-1640 medium supplemented with 10% (vol/vol) fetal bovine serum. THP-1 cells were primed with PMA (100 nM) for 3 h, washed three times and cultured overnight in serum-free DMEM medium. The cells were then stimulated with either liposomes or crystals for 18 h, and the supernatants were collected for the detection of human IL-1β by enzyme-linked immunosorbent assay (ELISA). BMDMs were generated by culturing the mouse bone marrow cells in the presence of 20% vol/vol L929 conditional media as previously described [12] , [53] . After pretreatment with ultrapure LPS (100 ng ml −1 for primary BMDMs and 50 ng ml −1 for immortalized macrophages) for 16–18 h, the BMDMs were stimulated with ATP for 30 min unless otherwise indicated or liposomes, alum, silica, MSU crystals or H 2 O 2 for 6 h. Poly(dA:dT) was transfected into the macrophages using Lipofectamine 2000 (4 μg ml −1 ) according to manufacturer’s instructions. For the experiments using chemical inhibitors, the inhibitors were added 45 min before stimulation with the NLRP3 inflammasome agonists. The blockade of potassium efflux with a high concentration of KCl was performed as previously described [9] . For the experiments using calcium-free medium, BMDMs were first primed with LPS for 18 h in calcium-containing DMEM, washed four times with PBS and then cultured in calcium-free DMEM in the presence of inflammasome agonists. Supernatants and cell lysates were collected for ELISA and immunoblotting analyses. Immortalized murine macrophages from Nlrp3 −/− , Asc −/− , Caspase 1 −/− , Nlrc4 −/− , Cathepsin B −/− , Aim2 −/− mice and their corresponding wild-type control cells were generously provided by Dr Katherine Fitzgerald and as previously described [12] . Enzyme-linked immunosorbent assay Paired (capture and detection) antibodies and standard recombinant proteins for mouse IL-1β, TNF and IL-6 (from eBioscience) were used to quantify the cytokine levels in cell culture supernatants according to the manufacturer's instructions. Mitochondrial ROS detection Mitochondrial ROS levels were measured using MitoSOX (Invitrogen). Briefly, LPS-primed cells were treated with liposomes for 6 h, loaded with 4 μM of MitoSOX for 15 min and washed twice with sterile PBS. The mean fluorescence intensity was determined using a FACSCantoflow cytometer (BD Bioscience), and the data were analysed using FlowJo software (Treestar). Fluorometric measurement of [Ca 2+ ] i The [Ca 2+ ] i was measured in single cells as previously described [55] . Briefly, cells were loaded for 30 min at 37 °C with 2 μM fura-2 AM in Tyrode solution containing 138 mM NaCl, 2.7 mM KCl, 1.06 mM MgCl 2 , 1.8 mM CaCl 2 , 5.6 mM glucose and 12.4 mM HEPES (pH 7.4, adjusted with NaOH). The fluorescence emission at 510 nm of fura-2 excited at 340 and 380 nm was acquired and analysed offline with the NIS-Elements Advanced Research software package (Nikon) using an inverted Nikon Ti-E microscope equipped with a Xenon lamp (Hamamatsu), a 40 × 1.30 NA objective (Nikon) and an Evolve 512 EMCCD camera (Photomatrics). The EMCCD camera was cooled to −80 °C during imaging. Quantitative real-time PCR analysis RNA was isolated from murine bone marrow-derived macrophages and was reverse transcribed. Quantitative real-time PCR analysis was performed using the StepOnePlus Real-time PCR system (Applied Biosystems). All gene expression data are presented as the expression relative to HPRT1. The primer sequences are described in the Supplementary Information . In vivo mouse peritonitis model Peritonitis induced by the intraperitoneal injection of stimuli has been described previously [13] . Briefly, 6- to 8-week-old mice were intraperitoneally injected with 1 mg MSU crystals, DOTAP liposomes or 0.2 mg zymosan dissolved in 0.5 ml sterile PBS. Six hours after injection, the mice were killed by exposure to CO 2 and the peritoneal cavities were washed with 8 ml cold PBS. The recruited polymorphonuclear neutrophils present in the peritoneal lavage fluid were quantified by flow cytometry using the neutrophil markers Ly6G (BD Bioscience) and CD11b (eBioscience). The samples were acquired on a FACSCantoflow cytometer (BD Biosciences) and the data were analysed using FlowJo software (Treestar). Immunization Six- to eight-week-old mice deficient in TRPM2 or IL-1R and the corresponding wild-type controls were subcutaneously immunized with OVA alone (40 μg per mouse), OVA-encapsulated DOTAP liposomes or OVA mixed with LPS, and the animals were boosted once after 2 weeks. Ten days after the final immunization, the mice were killed by exposure to CO 2 and the immune sera from the periphery blood were isolated. Statistics All data are shown as mean±s.d. or mean±s.e.m. Statistical analysis was performed using a two-tailed Student’s t -test for all studies. For all tests, P -values <0.05 were considered statistically significant. How to cite this article: Zhong, Z. et al . TRPM2 links oxidative stress to the NLRP3 inflammasome activation. Nat. Commun. 4:1611 doi: 10.1038/ncomms2608 (2013).